Consumer co-evolution as an important component of the eco-evolutionary feedback Rapid evolution in ecologically relevant traits has recently been recognized to significantly alter the interaction between consumers and their resources, a key interaction in all ecological communities. While these eco-evolutionary dynamics have been shown to occur when prey populations are evolving, little is known about the role of predator evolution and co-evolution between predator and prey in this context. Here, we investigate the role of consumer co-evolution for eco-evolutionary feedback in bacteria–ciliate microcosm experiments by manipulating the initial trait variation in the predator populations. With co-evolved predators, prey evolve anti-predatory defences faster, trait values are more variable, and predator and prey population sizes are larger at the end of the experiment compared with the non-co-evolved predators. Most importantly, differences in predator traits results in a shift from evolution driving ecology, to ecology driving evolution. Thus we demonstrate that predator co-evolution has important effects on eco-evolutionary dynamics. Consumer resource interactions are important components of virtually all ecological communities and have been studied extensively as they may determine the stability and diversity of these communities [1] . Concentrating on these interactions a variety of intriguing temporal dynamics can be observed. Already for simple consumer resource communities consisting of only two interacting species, the resulting temporal dynamics can range from extinction over stable coexistence to stable (and chaotic) oscillations and even more complex dynamics [2] , [3] , [4] , [5] , [6] , [7] , [8] . These dynamics are determined by different ecological factors [1] and can be altered by evolutionary processes when the evolutionary change is sufficient enough [9] , [10] , [11] , [12] . Similarly, ecological changes have the ability to alter evolutionary dynamics and, in some cases, this can lead to reciprocal interactions between ecology and evolution, so called eco-evolutionary feedback dynamics [13] , [14] , [15] . During the last decade, the effects of ecological on evolutionary change (the eco→evo), and vice versa (the evo→eco), and in some cases reciprocal effects, have been documented in a variety of empirical systems: laboratory microcosms [10] , [16] , [17] , mesocosms and enclosures [18] , [19] , [20] , [21] , as well as field studies of Darwin’s finches [22] , fence lizards [23] , freshwater copepods [24] , [25] , Soay sheep [26] and butterflies [27] . However, a demonstration of a complete feedback loop between evolutionary and ecological dynamics in a single system is still rare (but see ref. 9 ). Many examples for contemporary rapid evolution under controlled conditions stem from studies with microbes, as they are easy to culture and manipulate, have short generation times and large population sizes. Several examples from microbial laboratory experiments show evolution in the prey (host) in response to predation (or parasitism) [28] , [29] , [30] , [31] . In some cases this evolutionary change has also been documented to directly affect the ecological dynamics [10] , [16] , [17] , [32] , [33] , [34] . In addition to the strong evidence that the prey or host populations can evolve adaptations, there are observations that exploiter species (predators or parasites) can evolve within ecologically relevant time scales [33] , [35] , [36] . Furthermore there is evidence that both the consumer and the resource species evolve; a defensive adaptation in the prey (host) is followed by counter adaptation in the predator (parasite), which then causes further adaptation in the prey and so on, leading to antagonistic co-evolutionary dynamics [37] . Thus, the fitness of victim species continuously changes and depends on the heritable traits of the exploiter species and vice versa. Despite an increasing number of studies on eco-evolutionary dynamics in consumer resource systems, studies rarely have investigated the potentially important role of co-evolution for eco-evolutionary dynamics. Understanding how rapid co-evolution in ecologically important predator and prey traits can interact with populations and community dynamics requires controlled experimental manipulation of heritable trait variation. This allows testing if differences in traits of predators and/or prey change ecological and evolutionary dynamics simultaneously. Herein, we study the role of co-evolution on eco-evolutionary community dynamics by conducting two experiments using microbial communities with one prey, the bacterium Pseudomonas fluorescens, and one predator, the ciliate Tetrahymena thermophila . To disentangle the role of co-evolution, we separate evolution in the predator and the prey by first evolving the predator under different conditions (selection experiment) and then test for the effects of the differently evolved traits in the predator on eco-evolutionary dynamics (eco-evolutionary experiment). In the selection experiment, we evolve predator lines to obtain predator populations differing in trait variation, that is, their evolutionary history; evolved (predators adapted to prey) and co-evolved predators (predators adapted to evolving prey). After this 100-day selection period (equal to hundreds of predator generations) in continuous cultures co-evolved predators adapted to be more efficient in their resource use, indicating the change of a key ecological trait in the predator–prey interaction. In the second experiment, we then test for the role of this trait variation for eco-evolutionary community dynamics in 28-day-long microcosm experiments (semi-continuous cultures). Therefore, we inoculate microcosms with monoclonal prey and predators with different evolutionary histories: co-evolved, evolved and stock (no adaptation to any prey type) predators. This time period is sufficient for prey evolution but based on our own observations (see below) and a previous study with the same system [38] , we conclude that Tetrahymena does not evolve in a way that would have impact on ecological dynamics within 28 days (that is, de novo mutations do not occur or do not reach high enough frequencies in the population). However, within the originally more diversified evolved and co-evolved predator populations from the selection experiments (we use the evolved population and not one individual clone), micro-evolutionary dynamics, that is, changes in genotype frequencies, might occur during the microcosm experiment. By following predator and prey densities (ecological dynamics) and prey trait values D (level of defence against consumption by the predator) over time (evolutionary dynamics), we find that predators’ co-evolutionary history affect both ecological and evolutionary dynamics as well as the interactions between these. Our results suggest that the predator co-evolution can qualitatively alter the eco-evolutionary feedback and have important effects on community dynamics. Predator selection history We selected for trait variation in the predator using 100 days of continuous culture where ciliates grew either together with Pseudomonas (adaptation to evolved prey, hereafter co-evolved predators), were fed with non-evolving Pseudomonas (adapted to naive prey, hereafter evolved predators), or axenically without any bacteria (no adaptation to any prey type, hereafter stock predators; see Methods). We found that co-evolved predators grew significantly better on naive and evolved prey compared with stock and evolved predators after 100 days of continuous selection ( Fig. 1a , analysis of variance (ANOVA), n =3, F 2.6 =6.56; P =0.031, homogenous subsets; Tukey HSD, a: P =0.783; b: P =0.075; Fig. 1b , ANOVA, n =3, F 2.6 =9.93; P =0.013, homogenous subsets; Tukey HSD, a: P =0.94; b: P =1.0). This shows that co-evolved predators were more efficient consumers of both naive and evolved prey types. As ciliates grew without any prey for 1 week (~7 generations) between isolation from the selection experiments and the growth assays, the observed changes in growth rates are the result of evolutionary adaptation, rather than a plastic response. 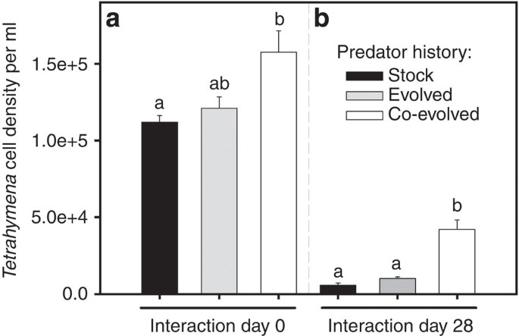Figure 1: Predator–prey interactions measured at the start and the end of the 28-day community experiment. (a) Effects of predator evolutionary history (after 100-day chemostat selection) on predator growth (final population density after 48 h) on ancestor naive prey. (b) Predator growth was measured again at the end of the 28-day community experiment with bacteria isolated from the microcosms (mean±s.e.,n=3). Letters (a or b) indicate subsets that are not different from each other. Figure 1: Predator–prey interactions measured at the start and the end of the 28-day community experiment. ( a ) Effects of predator evolutionary history (after 100-day chemostat selection) on predator growth (final population density after 48 h) on ancestor naive prey. ( b ) Predator growth was measured again at the end of the 28-day community experiment with bacteria isolated from the microcosms (mean±s.e., n =3). Letters (a or b) indicate subsets that are not different from each other. Full size image Ecological dynamics In a second set of experiments, we used the differently adapted predator strains to study eco-evolutionary dynamics in bacteria–ciliate communities. To ascertain that the predators were evolutionary stagnant during the following 28-day-long community experiment, we compared growth of the predators taken from the start and end of the experiment with stock predators. Stock predators were used to test the assumption that predator adaptation does not occur in 28 days, as they were the least adapted Tetrahymena strain to the bacterial prey. In a 48-h-long growth assay, where both predator lines were grown on evolved prey (taken from the end of the experiment) we found no difference between final population size of the predators isolated on day 0 and day 28 indicating that Tetrahymena co-evolution did not occur within 28 days (maximum cell density per ml for predators: isolated on day 0: mean±s.e. 4,666±933; isolated on day 28, mean:±s.e. 5,733±1,333, difference between two predators lines: ANOVA, n =3, F 1.4 =0.43; P =0.55). Comparing the population densities of the predator across the different treatments (stock, evolved, co-evolved predators) of the eco-evo experiment, we found that predators had on average higher densities in the co-evolved than in the stock treatment but not compared with the evolved treatment ( Fig. 2b–d , predator evolutionary history: repeated measures ANOVA (RMANOVA), n =3, F 2.6 =13.0; P =0.007, co-evolved and stock populations different at P =0.005 level; co-evolved versus evolved populations P =0.07, Tukey honest significant difference (HSD)). However, there were no significant differences in average prey population sizes ( Fig. 2b–d , predator evolutionary history: RMANOVA, n =3, F 2.5 =4.16; P =0.086). 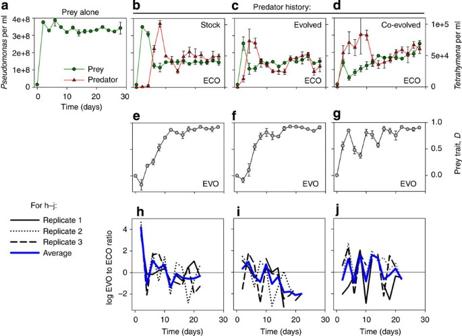Figure 2: Effect of predator treatment on ecological and evolutionary dynamics. Population densities over time: (a) prey alone; (b–d) predator+prey communities. Green lines presentP. fluorescensand red linesT. thermophilapopulation densities per ml (mean±s.e.,n=3). (e–g) Effect of predator treatment on evolutionary dynamics in prey level (mean±s.e.,n=3). (h–j) The relative importance of evolution (prey trait changeD) and ecology (prey density) to the predators’ growth rate in our predator–prey community. Inh–j, higher positive values onyaxis represent a situation when evolution is relatively more important than ecology and more negative values the opposite. Separate black lines represent individual microcosms in each treatment, blue line is the average of the three replicates and the vertical line is a reference line of 0, representing the level where evolution and ecology are equally important. No values are shown when ecological and/or evolutionary contribution was zero. Figure 2: Effect of predator treatment on ecological and evolutionary dynamics. Population densities over time: ( a ) prey alone; ( b – d ) predator+prey communities. Green lines present P. fluorescens and red lines T. thermophila population densities per ml (mean±s.e., n =3). ( e – g ) Effect of predator treatment on evolutionary dynamics in prey level (mean±s.e., n =3). ( h – j ) The relative importance of evolution (prey trait change D ) and ecology (prey density) to the predators’ growth rate in our predator–prey community. In h – j , higher positive values on y axis represent a situation when evolution is relatively more important than ecology and more negative values the opposite. Separate black lines represent individual microcosms in each treatment, blue line is the average of the three replicates and the vertical line is a reference line of 0, representing the level where evolution and ecology are equally important. No values are shown when ecological and/or evolutionary contribution was zero. Full size image Besides averaging over the whole 28 days, our experiment allows analysing changes in population sizes in more detail over time. We found significant differences in the initial population growth rates of the bacterial prey and its predator. Pseudomonas populations had the highest initial growth rates in the microcosm that were inoculated with stock predators and lowest in the microcosms started with co-evolved predators ( Fig. 2b–d , predator evolutionary history: RMANOVA, n =3, F 2.6 =13.5; P =0.006, co-evolved and stock populations different at P =0.005 level; co-evolved and evolved populations different at P =0.042 level, Tukey HSD). The pattern was reversed for the predator population growth rates ( Fig. 2b–d , predator evolutionary history: RMANOVA, n =3, F 2.6 =52.5; P <0.001, co-evolved and stock populations different at P =0.001 level; co-evolved and evolved populations different at P =0.034 level, Tukey HSD). Furthermore, the ratio of predator to prey, which is an estimate for species interaction strength, was initially higher in the populations that were started with co-evolved predator ( Fig. 3 ; days <10; predator evolution treatment: RMANOVA, n =3, F 2.6 =14.8; P =0.005, co-evolved and stock populations different at P =0.006 level and co-evolved and evolved populations different at P =0.012 level, Tukey HSD). This changed after the predator populations had reached their first maximum and after which predator/prey ratios were similar in all treatments ( Fig. 3 , days >10; predator evolution treatment: RMANOVA, n =3, F 2.6 =0.93; P =0.455). Although predator/prey ratios were not different after the first maxima, population densities were significantly elevated in predator and prey in the microcosms with co-evolved predators. Average prey population densities (±s.e.) days >10, in stock, 14.8±0.21 × 10 7 ; evolved, 14.7±0.37 × 10 7 and in co-evolved, 17.7±0.46 × 10 7 individuals per ml. ( Fig. 2b–d , days >10, effect of predator evolution treatment on prey densities: RMANOVA, n =3, F 2.5 =20.9; P =0.004, co-evolved and stock populations different at P =0.012 level and co-evolved and evolved populations different at P =0.004 level, Tukey HSD; and on predator densities: RMANOVA, n =3, F 2.6 =8.7; P =0.017, co-evolved and evolved populations different at P =0.015 level; co-evolved and stock populations different at P =0.085 level, Tukey HSD). 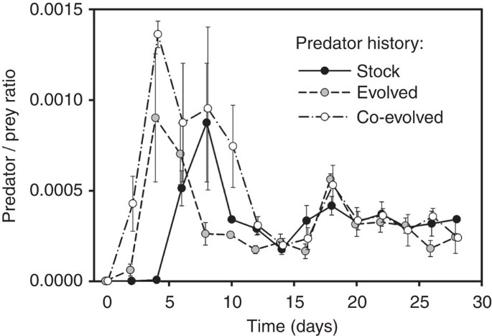Figure 3: Effect of predator history on predator to prey ratio. The figure shows ratios of densities (individuals per ml; mean±s.e.,n=3). Figure 3: Effect of predator history on predator to prey ratio. The figure shows ratios of densities (individuals per ml; mean±s.e., n =3). Full size image To further explore the role of co-evolution, we ran experiment using the stock predators but starting with evolved prey (evolved without predators; Fig. 2a ) and co-evolved prey (evolved with co-evolved predators; Fig. 2d ; both isolated at the end of the eco-evolutionary community experiment). We found that with evolved prey ( Supplementary Fig. 1a–c ), the community dynamics qualitatively followed the dynamics seen in the experiment with naive prey ( Fig. 2b ). However, with co-evolved prey, ciliates went extinct in two out of three replicates after two transfers ( Supplementary Fig. 1g–i ). Evolutionary dynamics Prey evolved efficient defences against ciliate predators during the 28-day-long community experiment within the first ~10 days ( Fig. 1 showing ciliate densities; difference between densities at day 0 and day 28, data pooled over the predator treatment: RMANOVA, n =3, F 1.22 =11.6; P =0.003; see Methods for measurements of defence levels). The predator evolutionary history had no effect on the average level of prey defences ( Fig. 2e–g predator treatment: RMANOVA, n =3, F 2.6 =2.39; P =0.17) as the prey defence reached similar levels in all treatments. We further tested for qualitative differences across treatments in the evolution of the prey defence. Compared with stock predators, initial prey adaptation was faster with co-evolved predators ( Figs 2e–g and 4a ; predator treatment RMANOVA, n =3, F 2.6 =11.9; P =0.008, homogenous subsets; a: P =0.204; b: P =0.062, Tukey HSD). The speed of adaptation in microcosms with evolved predators was similar to the rates of microcosms with stock predators. With co-evolved predators we also observed prey trait cycles that stabilized over time whereas no cycles were found in the other two treatments ( Figs 2e–g and 4b ; predator treatment: RMANOVA, n =3, F 2.6 =8.90; P =0.016, homogenous subsets; a: P =1.0, Tukey HSD). 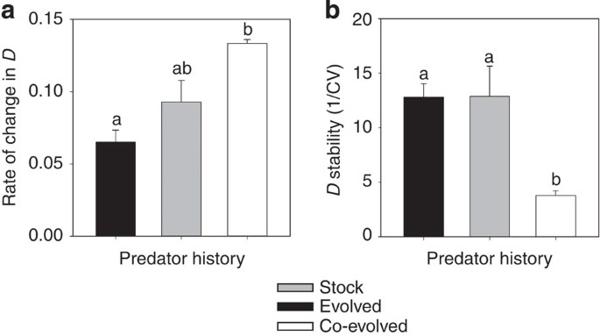Figure 4: Effect of predator history on the speed of initial adaptation in prey and the stability of the prey defence trait,D(mean±s.e.,n=3). Letters (a or b) within two variables indicate subsets that are not different from each other. (a) Rate of change in D, (b) stability ofD. Figure 4: Effect of predator history on the speed of initial adaptation in prey and the stability of the prey defence trait, D (mean±s.e., n =3). Letters (a or b) within two variables indicate subsets that are not different from each other. ( a ) Rate of change in D, ( b ) stability of D . Full size image In the experiment with co-evolved prey and stock predators ( Supplementary Fig. 1 ), we observed extinction of the predator in two out of three replicates with co-evolved prey indicated the higher level of prey defence of the co-evolved prey, which was confirmed by the measurements of the prey trait D ( Supplementary Fig. 1j–l ). The defence trait D evolved to lower defence levels after the predator went extinct In the other replicate, where predators and prey coexisted, the prey defence trait remained at a high level. With evolved prey, the defence trait rapidly increased to higher levels ( Supplementary Fig. 1d–f ), similar to the trait dynamics observed in the experiment with the naive prey and stock predators ( Fig. 2e ). Eco-evolutionary feedback We used cross correlations between the prey defence trait and the predator growth rate to further explore the observed ecological and evolutionary change over time and to link these. We would expect that there is a negative correlation between changes in the bacterial anti-predator defence and the predators’ population growth rates. We observed notable differences between the treatments with different predator evolutionary history ( Table 1 ). The predators’ growth rates were negatively correlated with a time lag of 2–6 days to the defence trait in the prey for stock predators, whereas there was no time lag between growth rate and the trait for evolved predators. For the co-evolved predators, the time lag was positive (4–8 days), that is, the predators’ growth was leading the trait evolution. Table 1 Summary of cross correlation analysis for the prey defence trait ( D ) and predator population growth rates. Full size table To further explore the role of ecology and evolution, we estimated the contribution of evolutionary and ecological change to the predators’ growth rate over time. The relative importance of changes in prey density and the prey defence trait can be partitioned through a two-way ANOVA [39] , [40] . As this method tests how the two processes affect changes in the predators’ population growth rate, rather than the absolute growth rate, we can use the ratio of the evolutionary to ecological contribution for comparison between treatments with different predator evolutionary history. These results are presented in Fig. 2h–j where positive values indicate that evolution is more important than ecology and negative values indicate that ecology is more important than evolution. The initial ratio (log of evo/eco) was positive for the stock predators, indicating that the evolutionary change in the prey population was more important than the change in the prey density at the beginning of the experiment. This changed after day 4 as there was only little change in the prey defence after this and predator population’s growth rates were mainly driven by ecological change, that is, prey density. The pattern was similar for the evolved predators. We found the opposite for the co-evolved predator treatments. Here, predators’ growth rates were initially driven by the change in prey densities (negative values), before the role of the evolutionary change in the prey population became more important. After this, the importance of ecology and evolution fluctuated. We experimentally studied how evolution in the consumer population affects ecological and evolutionary change in both the prey and predator populations. Using ciliates with different evolutionary history and thus traits affecting the predator–prey interaction, we found that the differences in species interaction altered the ecological as well as the evolutionary dynamics of the experimental predator–prey community. Altogether, our analysis shows that consumer evolution might have an important role in how ecological and evolutionary dynamics interact over time. A key finding when examining the ecological aspects of our experimental community was that both predator and prey populations reached higher population densities during the latter part of the experiment ( Fig. 2b–d : days 10 to 28) when started with co-evolved ciliates. This result indicates that co-evolution had important effects on long-term ecological dynamics and trophic interaction in our study system. Interestingly, however, our results suggest that differences in predator traits are a likely explanation for the elevated population sizes in both trophic levels with co-evolved ciliates, as the level of prey defence ( D ) reached similar levels in all treatments by the end of the experiment. Changing biomass or population densities as a result of rapid evolution and trait variation within the consumer populations have been shown in previous studies; Bassar and colleagues made similar observations as we when studying a number of ecological responses in mesocosm experiments with the Trinidadian guppy Poecilia reticulate [20] , [40] . They found that altered biomasses of several trophic levels depending on the evolutionary history of the guppies (individuals from high or low predation environments). Guppy evolutionary history had significant effects on, for example, algal stock, gross primary production and biomass-specific productivity. Another example comes from a series of studies by Post and colleagues who tested for eco-evolutionary dynamics resulting from an initial ecological change in planktivore fish populations (landlocking of populations that originally were able to migrate between freshwater and marine environments, that is, anadromous alewives, Alosa pseudoharengus ) [41] , [42] , [43] . Landlocked alewives exerted a constant grazing pressure on the zooplankton population throughout the year. Consequently, zooplankton population in these lakes evolved to be smaller and grew slower. These changes in zooplankton had in turn co-evolutionary consequences in the alewive feeding morphology (smaller gape width and gill-raker spacing) [44] , [45] . Modifications in zooplankton and alewife populations increased phytoplankton biomass and lowered net primary production. Conversely, anadromous alewife populations do not exert high grazing pressure throughout the year and thus have not caused and undergone the same evolutionary and ecological changes as their landlocked counterparts have. While the systems in these previous studies and in the present study differ in several ways (for example, food web structure and length, trophic cascades, nutrient recycling, number of generations followed in consumer population: less than one in the case of the guppies), it becomes clear that evolution and co-evolution on ecological timescales might be important for the flow of energy and matter through communities and food webs over time. In addition to evolution altering ecological dynamics and trophic interactions, we found evidence that altered ecological interactions impacted evolutionary change. Even though identifying the underlying mechanism of the higher rates of prey adaptation with co-evolved predators was not part of this study, we recognize that there are at least three non-exclusive mechanisms that could explain the differences in the initial pace of adaptation. First, grazing pressure by the co-evolved predator was higher compared with the evolved and in particular to the stock predators, resulting in higher selection pressure on the prey population. Second, the higher selection pressure led to smaller population sizes in the prey at the beginning of the experiment, which might have changed the relative importance of drift and selection and the supply of mutations [46] , [47] , [48] . A third explanation for the higher rates of adaptation with co-evolved predators is based on the observation of trade-offs between being defended and competitive. This trade-off has been demonstrated in several other experimental predator–prey systems [10] , [29] , [33] . When assuming an increasing cost with an increasing level of defence, a low level of defence will provide an advantage with stock and evolved predators, as they have no ability to overcome this defence. In contrast, the low level of defence will give you a disadvantage when growing with co-evolved predators as the predators have a counter-defence and the prey pays only the costs of the defence. As a consequence, the low and intermediate defended prey types are eliminated much faster from the prey population compared with the evolved and stock treatments, resulting in a faster increase in the level of defence of the population. More tests on the shape of the trade-off of being defensive and growth of the bacterial prey will be required as well as on the counter-defence mechanism of the ciliates (potential mechanisms are behavioural, morphological or physiological adaptations). In addition to effects of predator evolution on prey adaptation examined in here, previous studies have identified resource availability and temporal and spatial differences as important drivers for the co-evolutionary dynamics in host–parasite systems [35] , [36] , [49] as well as for prey evolution in predator–prey systems [29] , [33] . In our study, resources, that is, productivity was constant across treatments, but differences in traits of the predators had similar effects as differences in production: co-evolved predator populations increased rapidly at the beginning of the experiment resulting in high predator–prey ratios and higher encounter rates. Our main aim with this study was to explore feedbacks between ecological and evolutionary dynamics using a simple experimental predator–prey community. We found that our experimental treatment affected community dynamics in both ecological and evolutionary levels. We further tested for the interaction between ecology (predator population growth rate) and evolution (defence in the prey population) in more detail over time. When disentangling eco-evo feedbacks ( Table 1 , Fig. 2h–j ) we found that manipulating evolutionary history of the predator resulted in a shift from evolution driving ecology (stock predator), over ecology and evolution happening simultaneously (evolved predator; with the time resolution in the experiment) to ecology driving evolution (co-evolved predator). Similarly, the contribution of evolution (defence) was more important than ecology (prey density) for the predators’ population growth rate with stock predators, but the opposite was true for the co-evolved predators. The ‘pre-adaptation’ of the co-evolved predator probably allowed the predator to stay ahead of the evolving prey for a while until the higher levels of prey defenses evolved. In contrast, the stock predator's population growth rates were mainly driven by the evolutionary change in the prey population, as the predator had no ability to counter adapt. The temporal changes in importance of the ecological and evolutionary dynamics that we found here show in how many different and complex ways ecology and evolution can be entangled. Thus the rate of adaptation in the prey population was altered by changes in selection by the predator. This underlines the importance of species interactions as the ecological and evolutionary dynamics can have cascading and time-lagged effects within communities. More work is needed on the dependence of the rate of evolutionary change on the strength of selection, and how selection strength alters the potential and shape of eco-evolutionary dynamics [15] . Our findings support the general predictions from modelling and theoretical studies showing that increasing complexity (more interacting species and/or evolving traits) does not alter the potential for eco-evolutionary feedback dynamics [34] , [50] , [51] , [52] . Moreover, these eco-evolutionary dynamics with co-evolution should be highly relevant for the geographic mosaic of co-evolution [53] where temporal and spatial differences in the biotic and abiotic environment generate co-evolutionary mosaics, local adaption and range expansion [54] , [55] ), as well as for evolving communities [56] , [57] . In a full eco-evolutionary feedback loop, evolutionary processes significantly alter ecological dynamics and in return the altered ecological dynamics influence the evolutionary processes [13] . Our study demonstrates the interactions between the key components of an eco-evolutionary feedback loop on two trophic levels. We deliberately separated the evolutionary processes in the prey and predator population to gain a better understanding of the role of coevolution in eco-evolutionary dynamics. In the eco-evo experiment with stock and evolved predators, we showed the eco→evo→eco link, as grazing by the predator resulted in low population sizes, which further resulted in the evolution of a defence trait in the prey, lowering in return the predator densities (compared with the first maximum in the predator population size). The same was true for the experiments with the evolved prey and stock predators ( Supplementary Fig. 1a–c ). For the co-evolved predator, we started at different time point of the eco-evo feedback loop. Thus in the eco-evo experiment we observed the evo→eco→evo→eco link, when counting the co-evolution of the predator during the selection experiment as part of the feedback loop (co-evolved predators→reduction in prey population size→prey evolution→change in predator densities). An important observation is that in experiments with co-evolved prey and stock predators, previous evolution of high defence levels D resulted in a break of the eco-evolutionary dynamics as the predators could not counter adapt within the short timer-period. The next step to demonstrate a full eco-evolutionary feedback loop in this system requires that co-evolutionary and community dynamics studied simultaneously within one experiment. In addition to demonstrating the operation of the different links in an eco-evolutionary feedback loop in the experimental predator–prey community, our data illustrate the possibility that feedback loops might be transient. Another step necessary to better understand the role of co-evolution for eco-evolutionary dynamics is testing the effects of evolution in the prey and predator population in a full factorial design, that is, including treatments with evolved and co-evolved prey growing together with evolved and co-evolved predators. Importantly, and different from previous studies on co-evolutionary dynamics, we show here that prey adaptation and predator counter adaptation significantly alter the ecological and evolutionary trajectories. This can have significant consequences for the whole community when adaptation and counter adaptation are occurring at several trophic levels. In conclusion, considering evolution or trait variation at the consumer level and thus the potential for co-evolution adds another level of complexity for eco-evolutionary dynamics. Study system We used a well-established microbial system [28] , [30] consisting of one predator and one prey species. Our prey species was the heterotrophic bacterium P. fluorescens strain SBW25, originally isolated from a sugar beet leaf [58] . As a predator, we used the ciliated protist T. thermophila (CCAP strain 1630/1U). We followed standard protocols for microcosm experiments for this system. The culture media for bacteria contained M9 salts and King’s B nutrients in 5% concentration compared with the full strength media (concentrations used: 1 g Peptone number 3 and 0.5 ml glycerol in 1 litre of dH 2 O). We used PPY culture media containing 20 g of proteose peptone and 2.5 g of yeast extract in 1 litre of dH 2 O for growing Tetrahymena axenically (bacteria free). All culture media and microcosm were sterilized by autoclaving before use. Pseudomonas numbers were estimated as optical density (OD) at 600 nm wavelengths (UV-1800 spectrophotometer; Shimadzu, Japan). Optical density values were converted to cell numbers using the formula: cells per ml=OD × 8 × 10 8 . The conversion factor was determined by the standard curve method (OD versus CFU, colony forming units [59] ) from cells obtained from a steady state chemostat. We found that conversion between OD values and cell numbers was reliable within the range of OD values (~0.01–0.4) that we observed in the community experiment ( R 2 =0.998). Tetrahymena cell densities were enumerated directly from live samples using a compound microscope (Zeiss Axioskop 2 plus, Oberkochen, Germany). Selection for predators in continuous chemostat cultures To select Tetrahymena lines with different evolutionary histories we used 470-ml continuous culture chemostats maintained in growth chambers held at 28 °C (±0.1 °C). Setup and maintenance of chemostats followed the same methodology as in previous studies [10] , [16] , [60] , [61] . As a control for co-evolution we selected evolved predators, that is, predators adapted to feeding on naive prey, in a two-stage chemostat system. The first stage chemostat contained naive prey grown from a single smooth colony and the chemostat was fed with fresh culture media at the dilution rate of 0.2 per day. We then pumped prey from the first chemostat to the second-stage chemostat containing the predators (dilution rate of 0.1 per day), thus only prey individuals and no nutrients (since bacteria had consumed them completely) were transferred to the second stage. This prevented prey growth in the presence of predators and prey adaptation. As there was no prey adaptation to predation, co-evolutionary counter adaptations in predators were not expected. With this setup, the predators that had originally been maintained axenically in non-living peptone media, had a chance to adapt to feeding on live bacterial prey, making this a proper control for co-evolution experiments [62] . To our knowledge this is the first experimental co-evolution study with a predator–prey system where evolution control has been applied (see Table 1 in ref. 62 ). For selecting co-evolved predators, one single-stage chemostat was used and Pseudomonas and Tetrahymena were cultured together. The chemostat was fed with fresh culture media with the dilution rate of 0.1 per day. Constant input of fresh culture media allowed prey growth in the presence of predators and hence the evolution of a defence against consumption by the ciliate. On the basis of visual observation of large bacterial cell aggregates, a known defence mechanism against ciliated predators [63] , prey evolution occurred already after 7–10 days in response to ciliate predation. In return, the predator counter adapted to the prey defence ( Fig. 1 ). Both selection treatments were continued for 100 days and then predator cultures were made axenic again for the further experiments by incubating them in PPY growth media containing 500 units of penicillin per ml and 5 mg ml −1 of streptomycin for 24 h. This method obtained predator cultures with different evolutionary histories: co-evolved, evolved and stock predators. Eco-evo community experiment To experimentally test the effects of the predators’ evolutionary history on eco-evolutionary feedback dynamics, we conducted a 28-day-long microcosm experiment, representing ~160 prey and 90 predator generations. All treatments started from a single ancestor smooth colony of Pseudomonas (that is, there was no initial genetic variability in the prey population). For the different experimental treatments we started the microcosms with predator individuals having different evolutionary histories: co-evolved, evolved and stock predators. As control for the effect of predators we grew prey alone. All treatments were replicated three times in 25 ml glass vials containing 6 ml of 5% King’s B media. Every 48 h, 2.5% of each culture was transferred into a new vial containing fresh culture media. Microcosms were kept at 28 °C (±0.1 °C) with 50 r.p.m. constant shaking. During each transfer both predator and prey abundances were estimated and a 0.5 ml subsample was frozen with 0.5 ml of 80% glycerol and kept at −80 °C for later analysis. Ciliates do not survive freezing under these conditions. Experiments with evolved and co-evolved prey Following the eco-evo community experiments with naive prey and the different predator lines, we started further experiments with evolved and co-evolved bacteria. Therefore, we isolated Pseudomonas populations from the evolved (prey evolved without predators; Fig. 2a ) and co-evolved (prey evolved with co-evolved predators, Fig. 2d ) treatments and restarted the experiments with non-evolved stock predators (see above). Population were initiated and maintained with the same procedures as described above and terminated after five transfers. Measuring evolutionary changes in prey Evolution in the prey’s anti-predatory defence traits was analysed with a simple ecologically relevant bioassay. After thawing the samples from the eco-evo community experiment, a small subsample (100 μl) of each vial was used to inoculate 6 ml of fresh 5% King’s B, which was then maintained for 24 h at 28 °C (±0.1 °C). During this time all populations reached similar bacterial densities. Twenty-four hours correspond to more than 10 bacterial generations, indicating that phenotypic differences result indeed from evolutionary change rather than some induced defence mechanism. From the 6 ml cultures, a 100 μl sample was used to inoculate 2 ml of fresh 5% King’s B in 24-well plates. At this point, each well contained a prey population with different evolutionary history, obtained from the eco-evolutionary experiment. We then added 100 μl of stock predator containing 2,100 individuals into each well, that is, we used the naive stock predator as the ‘benchmark’ for consumer feeding on genetically differentiated prey. Before adding ciliates, high concentration PPY culture media was removed with centrifugation (3,000 r.p.m., 8 min, 4 °C) and the remaining pellet containing the ciliate cells was re-suspended in 5% King’s B. After 48 h, predator numbers were counted and the differences in final predator densities were then taken as an estimate for the prey defence levels [30] . This approach gives also direct (and relevant) information about the strength of the trophic link between prey and predator. Furthermore, since each well plate contained the ancestral prey as a control, we were able to compare each evolved prey population against the non-defended prey clone. Prey defence trait values were calculated as relative fitness by , where prey evo is the predator density fed on evolved prey, and prey anc the predator density when fed on the ancestral prey. Negative values or values close to zero indicate no or only a small difference in the defence level of the evolved prey compared with the ancestor prey. A value close to 1 means a high level of defence. Testing the effect of chemostat selection on predator When estimating the effects of long-term chemostat selection on predator co-evolution (data in Fig. 1 ) we used the same method as described above, with the exception that the evolutionary history of the predators was not uniform, that is, we used stock, evolved and co-evolved predator. Predator–prey interaction strength was quantified as differences in predator densities grown on different prey types for 48 h. Before these measurements, predators were cultured without the prey in axenic PPY culture media for one week, corresponding to several predator generations. Speed of adaptation and stability of prey trait dynamics The speed of initial adaptation in prey was calculated as the slope of log-transformed prey defence trait ( D ) data between the initial minima and the first maxima (see Fig. 2e–g ). For stock predators we used data from day 2 to day 12; evolved: day 2 to day 8 in two replicates and in one replicate day 2 to day 10; co-evolved predators day 0 to day 4. The stability of the trait dynamics was calculated as the inverse coefficient of variation (1/CV) between the first maxima and the end of the data set. Data analyses The effect of predator evolutionary history on growth rates was analysed with a two-way ANOVA. Post hoc Tukey HSD comparisons were performed to test for pairwise interactions. In the community experiment, the effect of predator evolution (treatment) on prey population densities and evolutionary change was analysed with repeated measurements ANOVA (RMANOVA) after log transforming the population density data. ANOVA analyses were performed with PASW statistics (SPSS Inc. Chicago, IL, USA v. 20.0) software. Sample size of three, used throughout the experimental procedure, was chosen on the basis of the high repeatability observed in the previous experiments. Rate of change in population size and change in the prey defence trait were calculated as r =ln( N t +1 / N t )/ t where N t is population size/trait value D at time t . Cross correlation analysis between predator population growth rates and prey defence traits were carried out in R statistical environment [64] . In addition, we used the Geber method described in Hairston et al. [39] to quantify the contribution of evolution (prey defence trait) and ecology (prey density) to the predators’ growth rates. The Geber method formalizes the idea that increases in the prey defence level and decreases in the prey density are predicted to have a negative influence on the predators’ growth rate. Full detail and description of the method can be found in Hairston et al. [39] How to cite this article: Hiltunen, T. et al. Consumer co-evolution as an important component of the eco-evolutionary feedback. Nat. Commun. 6:5226 doi: 10.1038/ncomms6226 (2014).